Engineeringp-wave interactions in ultracold atoms using nanoplasmonic traps Engineering strong p -wave interactions between fermions is one of the challenges in modern quantum physics. Such interactions are responsible for a plethora of fascinating quantum phenomena, such as topological quantum liquids and exotic superconductors. Here we propose a method to generate these fermionic interactions by combining recent developments in nanoplasmonics with progress in realizing laser-induced gauge fields. Nanoplasmonics allows for strong confinement, leading to a geometric resonance in the atom–atom scattering. In combination with the laser coupling of the atomic states, this is shown to result in the desired interaction. We illustrate how this scheme can be used for the stabilization of strongly correlated fractional quantum Hall states in ultracold fermionic gases. Recently, there has been growing interest in plasmonic nanostructures that can be used for various applications in quantum optics and atomic physics [1] , [2] , [3] , [4] , [5] , [6] , [7] . Of particular interest is the possibility of confining atomic motion over regions in space of order of nanometres, comparable or smaller than typical values of the atom–atom scattering length. In such a regime, atomic scattering undergoes strong modifications due to confinement-induced resonances [8] , [9] , [10] . Experimental difficulties to provide transverse confinement on the order of the atom–atom scattering length are surmountable, thanks to the new developments in plasmonics. A notable feature of surface-plasmon excitations, which exist along a metal–dielectric interface, is the lack of a diffraction limit. In the context of atom trapping, this enables the generation of fields with dramatically reduced effective wavelengths compared with free space, and a corresponding reduction of parameters, such as trap confinement. The properties of the plasmons can also be greatly engineered through the underlying device geometry. The interaction between Bose–Einstein condensates and tailored plasmonic micropotentials has recently been observed [3] , and plasmon-based trapping techniques for ultracold atoms with applications in quantum simulation have been proposed [1] , [2] , [4] . Here we propose to use nanoplasmonic trapping to engineer strong and robust p -wave interactions between fermionic atoms in planar geometries, which overcomes the challenges associated with creating such interactions with previously proposed techniques. This opens a new path towards the realization of exotic fractional quantum Hall states [11] , [12] and superfluid phases [13] , [14] . A strong motivation for realizing such states are their intriguing topological properties, which find direct application in topological quantum computation, protected quantum qubits and protected quantum memories [15] . Similarly, p -wave repulsion can stabilize low-filling fractional quantum Hall states [11] , [16] , including the Moore–Read state [12] . This state has been proposed in the context of a pronounced fractional quantum Hall plateau at filling 5/2 (ref. 14 ), but formally it also resembles the spinless chiral p -wave superfluid state. In solid-state physics, the most prominent example of p -wave superfluidity occurs in liquid 3 He (refs 17 , 18 ). Recently, also in strontium ruthenate, chiral ( p x + ip y )-wave Cooper pairs are believed to be responsible for the observed superfluidity of electrons [19] . In the field of quantum gases, strong p -wave interaction can in principle be achieved by using Feshbach resonances. Because of the inelastic loss processes, however, a strong p -wave interaction is hard to achieve experimentally [20] , [21] , [22] . Moreover, in Bose–Fermi mixtures, density fluctuations of bosons can induce attractive p -wave interactions or even higher partial waves between the fermions [23] , [24] , [25] . However, such proposals also run into difficulties due to the phase separation instability of Bose–Fermi mixtures and stringent constraints on temperature. Here we combine two important concepts: (1) strongly confined two-dimensional (2D) traps via nanoplasmonic fields and (2) strong laser-induced synthetic gauge fields as illustrated in Fig. 1 . For simplicity, the synthetic gauge field is produced through a minimal scheme described in ref. 26 . It consists of a laser field, coupling two internal levels of the fermionic atoms, and an external electric or magnetic field, which produces a linear variation of the energy of the internal states throughout the sample. Preparing the system in the lower-dressed state, the sample is effectively subjected to a strong synthetic magnetic field [27] . Being polarized in one dressed state, interactions between the fermionic atoms are prohibited by the Pauli principle. However, the external degrees of freedom provide a small coupling to the higher-dressed state. Remarkably, this will be shown to result in a residual p -wave contact interaction between the fermions, analogous to the synthetic higher partial waves reported in ref. 28 . This contribution can be enhanced, thanks to the resonant behaviour of the atom–atom scattering length in strongly confined 2D settings [9] , [10] as demonstrated recently in ultracold atomic systems [29] , [30] , [31] . This not only allows to strengthen the interaction but also to explore both attractive and repulsive p -wave interactions, that is, going from the physics of p -wave pairing to fractional quantum Hall physics. As a straightforward application of the scheme, we will consider the case of repulsive interactions and show by exact diagonalization how the induced p -wave interaction can be used to explore different quantum Hall phases, notably going from filled Landau level (LL) physics to the fractional quantum Hall regime with a ν =1/3 Laughlin state [11] , passing through a phase with sizable overlap with the Pfaffian state [12] . 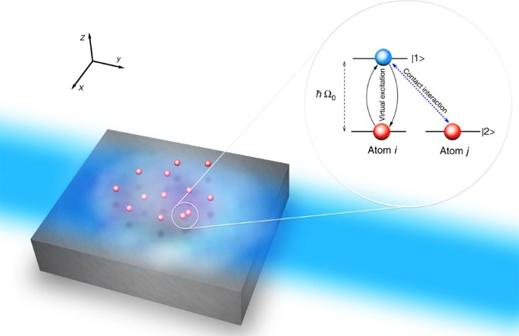Figure 1: Schematic depiction of the proposed setup. The ultracold atomic sample is tightly confined above a metallic surface as explained in detail in the Methods section. A laser beam (in blue), shining in from the side, is used to generate the artificial magnetic field felt by the atoms. The mechanism for fermion–fermion contact interaction involves the virtual excitation of one of the atoms into the excited dressed state, as illustrated in the inset. Figure 1: Schematic depiction of the proposed setup. The ultracold atomic sample is tightly confined above a metallic surface as explained in detail in the Methods section. A laser beam (in blue), shining in from the side, is used to generate the artificial magnetic field felt by the atoms. The mechanism for fermion–fermion contact interaction involves the virtual excitation of one of the atoms into the excited dressed state, as illustrated in the inset. Full size image Generation of the artificial magnetic field We consider a trapped ultracold gas of fermionic atoms with two internal states | g ,| e . The single-particle Hamiltonian H sp = H ext + H AL consists of an external part H ext = p 2 /(2 M )+ V ( r ) with the anisotropic trapping potential V ( r ) and an atom–laser coupling H AL , including also the internal energies. This coupling is responsible for a synthetic gauge field, which emerges due to the accumulation of Berry’s geometrical phase when an atom moves within the laser field [32] . The key to achieve non-vanishing phases on closed contours is to make the internal energies, and thus H AL , spatially dependent via a Stark or Zeeman shift, such that H AL and H ext do not commute (see Methods). The laser light mixes the ground and excited state, giving rise to position-dependent dressed states, |Ψ 1 and |Ψ 2 , which are the eigenstates of the atom–laser interaction (see Methods section for their explicit form). As detailed in the Methods section, increasing the laser strength, and thus the Rabi coupling between the two bare states, one can energetically favour one dressed manifold, say |Ψ 2 . By adjusting the external trapping, the single-particle Hamiltonian projected in this lowest dressed manifold can be written as the usual quantum Hall one, where ω ┴ is the effective xy trapping frequency, where and η is the strength of the synthetic gauge field, which depends on the laser wavenumber k and the spatial extent of the Stark or Zeeman shift w (see Methods). This Hamiltonian has the well-known LL structure, and its eigenfunctions are the Fock–Darwin states. Restricting ourselves to the lowest LL, the corresponding wave functions read where z = x − iy describes the atom position in the ( x , y ) plane. The adiabatic approximation requires large Rabi frequencies ħΩ 0 >> E R (ref. 27 ), where the recoil energy is . Within this limit, the off-diagonal Hamiltonian elements, H 12 and H 21 , connecting the dressed states are neglected. The explicit expression for H 12 is provided in the Methods section. Then, transitions to the higher-dressed manifold are fully suppressed. A general atomic state, becomes a low-lying solution for and . In our approach, however, some amount of non-adiabaticity is crucial, as it will yield a finite value for resulting in non-zero contact interactions. p -wave fermion–fermion interaction Now we turn to the atom–atom interactions, which we take as contact interactions. In terms of the bare fermionic states, it reads Here g c is a number quantifying the interaction strength. A more precise definition will be given later. Of course, in the dressed basis the interaction term maintains its form such that interactions remain restricted to pairs of one atom in |Ψ 1 and the other in |Ψ 2 . Thus, by polarizing the system in the lower-dressed state |Ψ 2 , no interactions are present in the adiabatic limit Ω 0 →∞. Still, by making the ratio of the Rabi frequency to recoil energy much bigger than 1, R E ≡ħΩ 0 / E R >>1, we can work in a quasi-polarized regime in which the |Ψ 1 level serves only as a virtual manifold. In this limit, the unperturbed many-body Hamiltonian is given by where the operator P i =|Ψ 2 i Ψ 2 | i projects the i th particle onto the low-lying Hilbert space. The off-diagonal terms, H 12 |Ψ 1 Ψ 2 | and H 21 |Ψ 2 Ψ 1 |, and the atom–atom interaction of equation (2) are taken as perturbations. They give second-order corrections. The effective many-body Hamiltonian can then be written as Note that the denominator in H (1) has been set to a constant equaling the energy difference between dressed states |Ψ 2 and |Ψ 1 . As this is taken to be large, it is the dominant contribution to the energy gap. In a previous study of a bosonic system [27] , [33] we have analysed the influence of H (1) , but the many-body contribution H (2) has been negligible because of the bosonic nature of the atoms. We will, in the following, show that in the fermionic case, where H (2) is the only many-body contribution, it becomes crucial. As illustrated in Fig. 1 , H (2) describes a process where one atom is excited from |Ψ 2 to the virtual |Ψ 1 manifold, where it interacts with an atom in |Ψ 2 , to then get de-excited to |Ψ 2 again. Importantly, acting among fermions the many-body interaction term gives solely non-zero p -wave contributions. This is seen by using equation (15) to cast H (2) into p -wave form (cf. ref. 16 ), with the relative variables, and z ij = z i − z j . The important feature of equation (4) is that the effective interaction is linear in the bare one, V ij , which allows one to change the interaction from attractive to repulsive. This is in contrast to second-order mechanisms like the Kohn–Luttinger [34] . The question that arises at this point is whether the interaction term, equation (5), is strong enough to significantly modify the physics of the system. This becomes possible by tuning the interaction strength g c . It is well known that this parameter crucially depends on the geometry of the system. In particular, for transversal confinements of the order of the scattering length, and considering the case of attractive interaction the effective 2D coupling is known to behave as [9] , [35] where ε is the energy of the motion in the x − y plane and a 3D the 3D (three-dimensional) scattering length. For a value of ħ ω z / ε =10 3 , it produces a resonant behaviour for values of the transverse confinement λ z ~0.4| a 3D |. Such confinement-induced resonance behaviour has been observed in experiments with optical traps by increasing the scattering length by means of Feshbach resonances [29] , [30] , [31] . This procedure, in particular if an optical Feshbach resonance is involved, suffers from severe loss processes. Approaching the shape resonance by decreasing the confinement length should minimize losses to the inevitable ones due to inelastic scattering of two particles. A candidate species for the gauge field proposal is ytterbium with narrow 1 S →3 P transitions. In this case, the loss rates for inelastic scattering between 1 S 0 and 3 P 2 can be minimized if spin-changing collisions are avoided by choosing the m =−2 hyperfine state [36] . With optical traps, the trapping on the z direction is usually of the order of hundreds of nanometres far from the resonance region. Nanoplasmonic trap properties The transverse confinement lengths of λ z ~5–10 nm needed to facilitate significant interactions can be achieved using novel plasmon-based trapping techniques, such as those investigated theoretically and experimentally in refs 1 , 2 , 3 , 4 . In the following, we present a detailed rendition of a hybrid plasmonic trap formed near a metal–vacuum interface. The stable trapping potential is formed by the combination of attractive Casimir–Polder forces (see Methods) and a repulsive barrier formed by blue-detuned surface plasmons (see Methods) guided along the interface. Below we show how this scheme can produce a transversal confinement of ~10 nm for a realistic implementation in the appropriate range to hit the confinement-induced resonance. This resonant behaviour can in principle be used to produce large values of g c and, importantly, also provides a way of producing both attractive and repulsive p -wave interactions between the fermions. Specifically, we consider surface plasmons propagating along an interface (at z =0) between vacuum ( z >0) and a metallic slab ( z <0), as illustrated in Fig. 4a. We assume that the surface plasmons are driven at frequency ω L > ω eg , where ω eg is the frequency of the atomic trapping transition. In this case, an atom near the surface experiences an optical dipole potential of the form , where corresponds to the transverse confinement length of the evanescent surface-plasmon field (see Methods). Here Ω is the corresponding Rabi frequency of the surface-plasmon field at the surface, and Δ= ω L − ω eg is the field detuning. Here we have assumed that Δ>>Ω, Γ, where Γ is the surface-modified excited state spontaneous emission rate. For positive detuning, the atom is repelled from the surface. In combination with the attractive Casimir–Polder potential (see Methods), the atom sees a total potential In certain parameter regimes, this can exhibit a meta-stable trapping potential, as illustrated in Fig. 2 , with the position of the local trap minimum given by z t . The presence of the optical field also gives rise to spontaneous photon scattering, at a surface-modified rate . As in conventional optical dipole traps, the effects of spontaneous scattering can be reduced by operating at large detunings and large intensities, as the scattering rate decreases with detuning at a higher rate than the optical dipole potential. 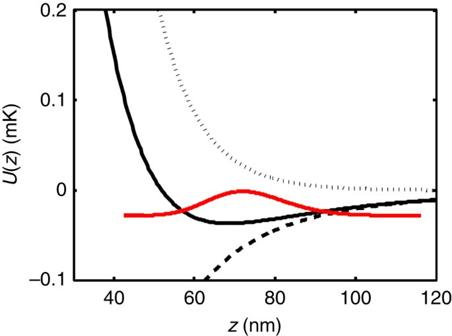Figure 2: Nanoplasmonic trapping potential. Total potentialU(z) (solid black curve), seen by the atom, versus distance to the metal interface. The contributions of the vacuum force (dashed curve) and of the repulsive plasmonic barrier (dotted) are also shown. The red curve depicts the ground-state wave function of the trap (in arbitrary units), which for the chosen parameters is localized to Δz=10 nm. Figure 2: Nanoplasmonic trapping potential. Total potential U ( z ) (solid black curve), seen by the atom, versus distance to the metal interface. The contributions of the vacuum force (dashed curve) and of the repulsive plasmonic barrier (dotted) are also shown. The red curve depicts the ground-state wave function of the trap (in arbitrary units), which for the chosen parameters is localized to Δ z =10 nm. Full size image In the case of a plasmonic trap, the maximum detunings and intensities will in practice be dictated by residual optical absorption and the subsequent material heating. Specifically, the imaginary part of the material electric permittivity ε ( ω ) gives rise to a local energy absorption per unit volume and per unit time, , where E 2 is the electric field of the surface plasmons in the metal. Given the tight localization of the surface plasmons near the surface, we can approximate the heating as a delta function source, where accounts for the total energy absorption per unit area and per unit time in the metal. The temperature rise of the metal is then governed by the heat equation including the source, . Here c V is the heat capacity of the metal per unit volume and α is the thermal diffusivity. Assuming that the trap is turned on at t =0, the maximum temperature increase (which occurs at the interface z =0) is given by As a specific example, we consider the trapping of Yb atoms using the strong 6 s 2 -6 s 6 p transition, which has a resonant wavelength of λ 0 =399 nm and a spontaneous emission rate of Γ 0 =2π × 29 MHz. We use a Drude model for the optical response of the metal, where ω p and γ describe the plasma frequency and dissipation rate, respectively. We take material parameters of α =1.66 × 10 −4 m 2 s −1 , c V =2.44 × 10 6 J m −3 K −1 and , which correspond closely to silver. Note that choosing a particular material fixes the plasmon frequency, whereas ideally this should be a tunable parameter (such that the laser detuning Δ and surface-plasmon wavelength can be independently tuned). It is well known that changing the material geometry from the thick membrane considered here enables such tuning. To facilitate theoretical analysis, however, we restrict ourselves to the case of a thick membrane and assume that ω p is variable. As described above, we specifically target trap parameters such that the ground-state wave function of the trap has a position uncertainty of Δ z <10 nm, with the maximum possible detunings and intensities to minimize spontaneous photon scattering and before heating of the material becomes important on time scales relevant to the experiment. In the case of the parameters above, we find that this can be achieved by choosing atom-trapping parameters Ω/Γ 0 ~3 × 10 3 and Δ/Γ 0 ~5 × 10 5 , and material parameter (yielding a surface-plasmon wavelength of λ SP ~120 nm). The trapping potential for these parameters, along with the ground-state wave function, is illustrated in Fig. 2 . For these parameters, we find a scattering rate of R sc ~2π × 3 Hz, a ground-state uncertainty of Δ x ~10 nm and the trap potential minimum located at z t =70 nm from the metal surface. For these parameters, the trap can be sustained for approximately t ~100 ms without adverse effects from material absorption and heating. Stabilization of the ν =1/3 Laughlin state As an example, we discuss the case of repulsive p -wave interaction. In the context of quantum Hall physics we have to ask whether the obtained p -wave interaction is capable of bringing the system from the integer quantum Hall regime of a non-interacting system to the fractional quantum Hall regime. In that case, a Laughlin-like state should show up as the ground state of the system. Let us recall the Laughlin wave function [11] at filling ν , which has well-defined z component of the angular momentum operator , where L z = ν −1 N ( N −1)/2. Note that in the quantum Hall regime, η →1, the contribution of H 22 reduces to a constant, as all Fock–Darwin states become (quasi)degenerate. Thus, to bring the system into the fractional quantum Hall regime the interaction term must be comparable to the contribution of the H (1) term, which breaks the rotational symmetry [33] . To give definite numerical predictions, we perform an exact diagonalization (see Methods) with a few number of atoms, N =4. The parameters of the system are taken as k =10/ λ ┴ , ħΩ 0 =100 E R and η =0.98. We discuss the different phases appearing as we vary the interaction strength, g c . For weak interactions, the ground state of the system has a large overlap with the analytical form of the filled LL state, ν =1, as depicted in Fig. 3 . The angular momentum of the ground state is found to be slightly larger than the analytical value, L =6. As explained in refs 27 and 33 , this is due to the deviation from rotational symmetry. When the interaction is increased, the system undergoes a transition into a phase, where the ground state has large overlaps with the fermionic Moore–Read state [12] . Even stronger interactions bring the system into a state, which resembles the quasiparticle excitation of the ν =1/3 Laughlin state. At another critical value of g c , one finally reaches a ν =1/3 Laughlin-like state. In particular, as shown in ref. 27 , despite the broken rotational symmetry, this state still possesses the typical features of the Laughlin states, namely strong anticorrelations exhibited in the pair-correlation function, in contrast to an almost homogeneous density. As in the case of bosons with contact interactions, these anticorrelations make it a state of zero interaction energy, and thus no more transitions take place when further increasing the interaction parameter. These properties can be used for an experimental detection of the phases and strongly influence also the dynamical behaviour of the system as discussed in ref. 37 . 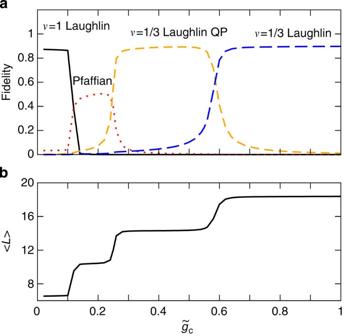Figure 3: Many-body quantum phases. Evolution of the ground state as a function of the interaction parameter. (a) The overlap fidelity, |Ψtarget|Ψgs| of the ground state with the filled LL state (solid black), the fermionic Pfaffian state (dotted red), the quasiparticle state over theν=1/3 Laughlin (dashed orange) and theν=1/3 Laughlin (long-dashed blue). (b) The average angular momentum of the ground state of the system. Figure 3: Many-body quantum phases. Evolution of the ground state as a function of the interaction parameter . ( a ) The overlap fidelity, | Ψ target |Ψ gs | of the ground state with the filled LL state (solid black), the fermionic Pfaffian state (dotted red), the quasiparticle state over the ν =1/3 Laughlin (dashed orange) and the ν =1/3 Laughlin (long-dashed blue). ( b ) The average angular momentum of the ground state of the system. Full size image We have presented a novel mechanism to realize sizable p -wave interactions between fermionic atoms. The key is the combination of a strongly confining plasmonic field, which allows to explore confinement-induced resonances, with a simple scheme to generate a strong synthetic gauge field. To exemplify the potential of our approach, we have considered the case of repulsive p -wave interaction. We have shown that our proposal allows to stabilize a number of interesting quantum Hall states, such as the Pfaffian, and the ν =1/3 Laughlin state. In our numerical calculation we have considered a small number of atoms, as it has become experimentally feasible recently [38] , [39] , [40] , but we note that the scheme should also be applicable to large systems. A good candidate for realizing the proposal are ytterbium atoms due to the long-lived state of the clock transition. Requiring an ultratight trapping in a 2D geometry, our proposal shall trigger the use of nanoplasmonic fields as a promising technique for achieving that goal. Single-particle Hamiltonian The single-particle Hamiltonian reads where H ext = p 2 /(2 M )+ V ( r ) with the anisotropic trapping potential V ( r ). H AL is the atom–laser coupling, which includes the internal energies. To make H AL spatially dependent, such that H AL and H ext do not commute, we perform a Stark or Zeeman shift of the internal energies. The strength of this shift can be characterized by a length scale w , which is chosen such that the energies of the bare internal states read E g =−ħΩ 0 x /(2 w ) and E e =ħ ω A +ħΩ 0 x /(2 w ). Here, ω A is the energy difference of the bare states. In this way, preparing the system in the ground state of H AL , the external part will stimulate transitions into the excited manifold of H AL . The probability of such transitions is controlled by the Rabi frequency Ω 0 of the coupling. The laser frequency is set to resonance with the atomic transition. Furthermore, we choose the laser to be a running wave in y direction with wavenumber k . Then, within the rotating-wave approximation, the atom–laser Hamiltonian H AL can be written in terms of bare states | e and | g as [41] where , tan θ = w / x , and φ = ky . Note that spontaneous emission processes are not considered in the Hamiltonian of equation (11). This is justified if the two atomic states are sufficiently long-lived, as is the case for the 1 S 0 → 3 P 0 clock transition in ytterbium. In contrast to the bosonic ytterbium isotopes, the finite spin of the fermionic isotopes yields a small magnetic moment, which allows for a strong coupling of the clock states at reasonable laser power. Thus, achieving large Rabi frequencies, as required by our proposal, poses no problem for 171,173 Yb (ref. 42 ). Diagonalizing equation (11) yields the dressed states, |Ψ 1 = e − iG ( Ce iφ /2 | g + Se − iφ /2 | e ), |Ψ 2 = e iG (− Se iφ /2 | g + Ce − iφ /2 | e ), where C =cos θ /2, S =sin θ /2, . The single-particle Hamiltonian H sp can be expressed as a 2 × 2 matrix H ij . In the dressed-state basis, its diagonal terms can be written as [27] with ε 1 =1 and ε 2 =−1. Full expressions for the vector potential A and the scalar potential U are given in ref. 27 . Note that for w << x , y , we recover the symmetric gauge expression . With a convenient choice of the trapping potential, H 22 can be made symmetric with respect to rotations around the z -axis. Then, the Hamiltonian element H 22 reads where ω ┴ is the effective xy trapping frequency, and . The recoil energy of the atoms is defined as . Retaining up to quadratic terms, the off-diagonal Hamiltonian elements, explicitly read with , , and . Acting on a Fock–Darwin state, the operators ( ) decrease (increase) the l quantum number by one, whereas the operators and change the LL. As we will be interested in the fractional quantum Hall regime of large synthetic magnetic field, , it is possible to safely neglect the and contributions. In this limit, we have and . In our numerics, we will furthermore choose and k =10/ λ ┴ , implying , guaranteeing c 1 << c 3 . We can then write Exact diagonalization To solve the effective Hamiltonian, we performed exact diagonalization. Therefore, we build many-body states using as single-particle states the Fock–Darwin states, | l . Then, the second quantized form of H (2) is where anihilates an atom in . The matrix element reads, V ij , kl =(ħΩ 0 ) −2 i | j | H 21 VH 12 | l | k . Taking into account the Pauli principle, we get where . With the expression for H 12 from equation (15), h l is directly found to be It is worth noting that due to the contact nature of the interaction, equation (16) commutes with . Casimir–Polder potential Here we provide a heuristic derivation of the Casimir–Polder potential for an atom in its electronic ground state, while referring the reader to ref. 43 for details. Working within a two-level approximation with atomic ground and excited states | g ,| e , the interaction between the electromagnetic field and an atom at position r is given by the dipole Hamiltonian H =− d . E ( r ). Following a complete decomposition of the electric field into its normal modes k , one can write . Here g k are the vacuum Rabi coupling strengths between the atom and mode k , and σ ij =| i j | are operators acting on the atomic internal states. The non-rotating terms of this Hamiltonian enable an atom in its ground state | g ,0 to couple virtually to the excited state and create a photon, | e ,1 k . The corresponding frequency shift for the ground state within second-order perturbation theory due to these quantum fluctuations is . This shift results in a position-dependent mechanical potential for the atom when translational symmetry is broken due to dielectric surfaces. A quantization scheme of the electromagnetic field in the presence of dielectrics in fact allows this expression involving the summation of modes to be conveniently rewritten in terms of the (classical) dyadic electromagnetic Green’s function evaluated at imaginary frequencies ω = iu , Here Γ 0 is the free-space spontaneous emission rate of the atom. The Green’s function is defined through the relation The shift δω g ( r ) is independent of the hyperfine or magnetic sublevel of the ground-state atom. As an example system, we consider the metal–vacuum interface shown in Fig. 4a . We treat the dielectric function of the metal as a Drude response, . Here ω p and γ characterize the plasma frequency and dissipation rate of the material, respectively. This dielectric function is a good approximation for metals, such as silver and gold. 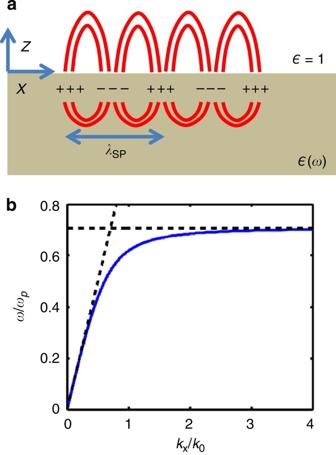Figure 4: Plasmon illustration. (a) A metal–vacuum interface (here, with interface located in thez=0 plane) supports guided surface-plasmon modes. These surface plasmons are a combined excitation of a charge density wave localized near the surface and an electromagnetic field (electric field lines depicted in red). The surface-plasmon wavelengthλSPand the transverse confinement of the mode can be reduced far below the free-space wavelengthλ0for frequencies whereε(ω)→−1−. (b) Blue curve: surface-plasmon dispersion relation,ωversuskx, in the case of the lossless Drude model. The diagonal dashed line indicates the free-space dispersionω=ck, whereas the horizontal line indicates the plasmon resonance frequencyabove which the the surface-plasmon modes are cut off. For atomic distances to the surface z << λ 0 that are much closer than the atomic resonant wavelength λ 0 , and for an atomic frequency comparable to the plasmon resonance frequency (where ε =−1), , equation (18) can be evaluated in the near field, Figure 4: Plasmon illustration. ( a ) A metal–vacuum interface (here, with interface located in the z =0 plane) supports guided surface-plasmon modes. These surface plasmons are a combined excitation of a charge density wave localized near the surface and an electromagnetic field (electric field lines depicted in red). The surface-plasmon wavelength λ SP and the transverse confinement of the mode can be reduced far below the free-space wavelength λ 0 for frequencies where ε ( ω )→−1 − . ( b ) Blue curve: surface-plasmon dispersion relation, ω versus k x , in the case of the lossless Drude model . The diagonal dashed line indicates the free-space dispersion ω = ck , whereas the horizontal line indicates the plasmon resonance frequency above which the the surface-plasmon modes are cut off. Full size image where k 0 =2π/ λ 0 is the resonant free-space wave vector. Although this asymptotic scaling is convenient to understand the trap properties, in numerical solutions presented later, equation (18) is evaluated exactly. In addition to the Casimir–Polder shifts, the metallic interface can also give rise to a modification of the excited-state spontaneous emission rate. Under weak driving by a laser of frequency ω L , a similar calculation shows that the effective spontaneous emission rate is given by Here the emission rate depends only on the Green’s function evaluated at the laser frequency, which reflects the interaction between the atom and its Rayleigh emission reflected from the metallic interface. Surface plasmons Surface plasmons are polaritonic excitations of an electromagnetic field and a charge density wave, which propagate along the surface of a metal–dielectric interface. Here we specifically consider surface-plasmon excitations at the metal–vacuum interface depicted in Fig. 4(a) . On the vacuum ( i =1) and metal ( i =2) sides, the electric fields are given by where and . Here, without loss of generality, we have considered excitations in the x – z plane. Enforcing proper boundary conditions of the field at the metal–vacuum interface, z =0, yields the dispersion relation for the surface plasmons and t =− k z / q z . It can be seen that as ε →−1 − , the in-plane wave vector k x diverges, leading to a very short surface-plasmon wavelength λ SP ≡2π/ k x . It also follows that the perpendicular component k z ≡ i κ z becomes large and imaginary, implying that the surface plasmons are tightly confined to the interface in the transverse direction. For the Drude model, this tight confinement occurs at frequencies near as illustrated in Fig. 4b . How to cite this article: Juliá-Díaz, B. et al . Engineering p -wave interactions in ultracold atoms using nanoplasmonic traps. Nat. Commun. 4:2046 doi: 10.1038/ncomms3046 (2012).